Visualizing autophosphorylation in histidine kinases Reversible protein phosphorylation is the most widespread regulatory mechanism in signal transduction. Autophosphorylation in a dimeric sensor histidine kinase is the first step in two-component signalling, the predominant signal-transduction device in bacteria. Despite being the most abundant sensor kinases in nature, the molecular bases of the histidine kinase autophosphorylation mechanism are still unknown. Furthermore, it has been demonstrated that autophosphorylation can occur in two directions, cis (intrasubunit) or trans (intersubunit) within the dimeric histidine kinase. Here, we present the crystal structure of the complete catalytic machinery of a chimeric histidine kinase. The structure shows an asymmetric histidine kinase dimer where one subunit is caught performing the autophosphorylation reaction. A structure-guided functional analysis on HK853 and EnvZ, two prototypical cis- and trans -phosphorylating histidine kinases, has allowed us to decipher the catalytic mechanism of histidine kinase autophosphorylation, which seems to be common independently of the reaction directionality. Post-transcriptional modification by phosphorylation is the most widespread mechanism in signal transduction. Transferring γ-phosphate from ATP to specific residues is the centrepiece in this process. In two-component systems, the main signal-transduction mechanism in bacteria, the signalling process starts by the autophosphorylation of a conserved histidine in the sensor histidine kinase (HK). Transfer of the phosphoryl group from the HK histidine to a conserved acid aspartic of its partner’s response regulator (RR) propagates the signal and triggers the cellular response [1] , [2] . Prototypical HKs are membrane-bound homodimers, which require two structurally conserved cytoplasmic catalytic domains to achieve autophosphorylation. One catalytic domain, named DHp (dimerization histidine phosphotransfer domain), is formed by two long helices (α1 and α2), where α1 contains a phosphorylatable conserved His residue. The second catalytic domain, named CA (catalytic ATP-binding domain), binds ATP in a pocket covered by a flexible and variable loop named ATP lid [3] , [4] . This domain displays an α/β sandwich fold similar to the ATPase domains of the GHKL (gyrase, Hsp90, histidine kinase, MutL) ATPase superfamily [5] . In orthodox HKs, DHp and CA are connected by a flexible and short (5–10 residues) loop. HKs function like dimers and dimerization takes place by the interaction of DHp helices to form a four-helix bundle. Autophosphorylation occurs when the ATP bound in CA phosphorylates the His in DHp. Yet, despite the different approaches used, a full structural characterization of the autophosphorylation reaction in HK remains elusive. This may be due to the highly dynamic nature of CAs, as demonstrated in DesK, HK853, VicK and YF1 HK structures, which can adopt different rearrangements [6] , [7] , [8] , [9] , [10] , [11] , and might also be due to the asymmetry in the autophosphorylation reaction, as proven for NRII [12] . The recent structures of VicK [9] and YF1 (ref. 8 ) HKs are consistent with the notion of asymmetry in the autophosphorylation reaction since these structures showed that one of the CA domain approaches to the phosphoacceptor His while the second CA domain is far away from the second His. Unfortunately, the absence of a nucleotide triphosphate in the catalytic centre of these structures has prevented the visualization of the autophosphorylation reaction. Flexibility and asymmetry, along with the transient nature of the intermediate state [ADP–P–His] in HKs [13] , have hampered the crystallization of a HK in the midst of the autophosphorylation reaction. Furthermore, HK dimerization implies that the directionality of the autophosphorylation reaction can either proceed in a cis - or trans -manner [7] , [14] , [15] . A cis -autophosphorylation reaction occurs by an intrasubunit manner; that is, the ATP bound in the CA domain of one subunit would phosphorylate the His in the DHp of the same subunit. In contrast, a trans reaction implies an intersubunit autophosphorylation. Biochemical data have confirmed the existence of both cis- and trans- mechanisms in different HKs [7] , [15] , [16] . Structural comparison of the DHp domains in HKs autophosphorylating in cis and in trans (data available from EnvZ and HK853 (refs 6 , 17 )) has provided some clues about the differences in the directionality of the autophosphorylation. The superposition shows that the loop connecting helices α1 and α2 in the DHp domain (DHp connector) has different handedness and length. We previously proposed that these differences can explain why a trans -mechanism in EnvZ corresponds to a cis -mechanism in HK853 (refs 7 , 18 ). Although structural confirmation of this hypothesis is still not available, recent biochemical results support this proposition. In that work, EnvZ was converted from a trans- to a cis- autophosphorylating enzyme by interchanging the α1–α2 DHp connector with the corresponding region of PhoR, a cis -autophosphorylating HK [19] . Here we provide a detailed analysis of the basis that lies behind the autophosphorylation mechanism in HKs by determining the structure of a chimeric EnvZ that incorporates the DHp connector of HK853. The structure shows a dimeric HK adopting an asymmetric conformation where one of the subunits is autophosphorylating. To decipher the HK autophosphorylation reaction, we perform a structure-guided functional analysis on residues in the active centre for HK853 and EnvZ, the models for cis - and trans -autophosphorylation. Thus, we evidence a reaction mechanism with a dissociative character where the nucleophility of the attacking His is activated by an acidic residue next to the phosphorylatable His, which acts as a general base and is assisted by a conserved polar residue in the CA domain. Meanwhile, the transferred phosphoryl group is stabilized by the main chain of a flexible conserved Gly-rich loop. This mechanism in HKs seems to be universal since it is conserved in both cis- and trans- autophosphorylating enzymes. Design and activity of HK853 and EnvZ chimeras The structural comparison of the EnvZ and HK853 DHp domains revealed two main differences; first, the handedness of the DHp connector between helices α1 and α2; second, the length of the DHp apex (eight residues shorter in EnvZ) ( Fig. 1a,b ). To get insights into the structural basis of an autophosphorylation reaction and to evaluate the contribution of the DHp connector in this reaction, we interchanged this region on the DHp apex between EnvZ and HK853 ( Fig. 1b ), which are two prototypical HKs with the trans - and cis -kinase mechanisms [7] , [16] . In EnvZ, residues from Leu254 to Tyr265 (LATEMMSEQDGY) were interchanged by HK853 residues from Ala271 to Glu290 (AYAETIYNSLGELDLSTLKE) to generate EnvZ chim ( Fig. 1b ). In the same way, HK853 residues from Ala271 to Glu290 were interchanged by EnvZ residues from Leu254 to Tyr265 to generate HK853 chim ( Fig. 1b ). To confirm the functionality of these chimeras, we examined their autophosphorylation capacities ( Fig. 1c ). EnvZ chim and HK853 chim showed similar phosphorylation rates as the corresponding wild-type EnvZ and HK853, thus confirming that swapping the DHp connector does not significantly affect the autophosphorylation reaction. 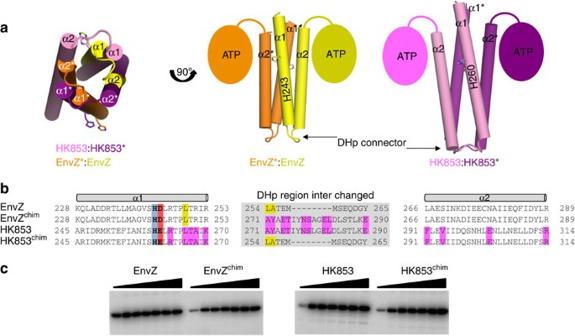Figure 1: Design and activity of HK853 and EnvZ chimeras. (a) Observation of the differential DHp connector handedness between EnvZ and HK853. Cartoon representation in cylindrical helices for the DHp superimposition of homodimeric HK853 (2C2A; one subunit in pink and the other (*) in purple) and EnvZ (3ZRW; one subunit in yellow and the other (*) in orange). A view of the independently superimposed structures rotated 90° is in the right side. In this view, the CA domain has been drawn connected to the α2 helices. The helices in the homodimers are labelled and phosphorylatable His is shown as sticks. (b) The DHp sequence from EnvZ, HK853 and the generated chimeras, EnvZchimand HK853chimare aligned and the DHp region interchanged to form chimeras is highlighted in grey. The phosphorylatable His is highlighted in blue and the acidic residue after the His is highlighted in red. Residues involved in RR recognition and binding in the HK853–RR468 complex are highlighted7in magenta and residues involved in rewiring phosphotransfer for EnvZ27are highlighted in yellow. (c) Autophosphorylation assays of HK853, HK853chim, EnvZ and EnvZchim. The HKs were incubated with [γ32]ATP for 1, 2.5, 5, 7.5, 10, 15 and 30 min at 37 °C. The phosphorylated proteins were visualized by autoradiography. Figure 1: Design and activity of HK853 and EnvZ chimeras. ( a ) Observation of the differential DHp connector handedness between EnvZ and HK853. Cartoon representation in cylindrical helices for the DHp superimposition of homodimeric HK853 (2C2A; one subunit in pink and the other (*) in purple) and EnvZ (3ZRW; one subunit in yellow and the other (*) in orange). A view of the independently superimposed structures rotated 90° is in the right side. In this view, the CA domain has been drawn connected to the α2 helices. The helices in the homodimers are labelled and phosphorylatable His is shown as sticks. ( b ) The DHp sequence from EnvZ, HK853 and the generated chimeras, EnvZ chim and HK853 chim are aligned and the DHp region interchanged to form chimeras is highlighted in grey. The phosphorylatable His is highlighted in blue and the acidic residue after the His is highlighted in red. Residues involved in RR recognition and binding in the HK853–RR468 complex are highlighted [7] in magenta and residues involved in rewiring phosphotransfer for EnvZ [27] are highlighted in yellow. ( c ) Autophosphorylation assays of HK853, HK853 chim , EnvZ and EnvZ chim . The HKs were incubated with [γ 32 ]ATP for 1, 2.5, 5, 7.5, 10, 15 and 30 min at 37 °C. The phosphorylated proteins were visualized by autoradiography. Full size image Structure of EnvZ chim To gain insight into HK autophosphorylation, we solved the crystal structure of EnvZ chim in the presence of the non-hydrolysable ATP analogue AMPPNP. The EnvZ chim structure was determined by single isomorphous replacement combined with anomalous scattering (SIRAS) using the diffraction data from a native crystal (3.0 Å) and a selenomethionine-substituted derivative (3.8 Å) crystal ( Table 1 ). The asymmetric unit of the crystal contained two EnvZ chim subunits forming the prototypical HK dimer by the interaction of the DHp domains ( Fig. 2a ) with all residues well defined in the electron density ( Supplementary Fig. 1 ), except for the first 7 (224–230) and the last 10 (441–450) residues. Comparison of the DHp four-helix bundle of the EnvZ chim dimer with the corresponding regions of EnvZ and HK853 revealed that the α1–α2 connection matches that observed in HK853 ( Fig. 2b ). Indeed, the EnvZ chim four-helix bundle superimposed better with HK853 than with EnvZ (r.m.s.d. 1.6 versus 3.0 Å), although only 19 out of 73 residues of DHp domain belonged to HK853. This observation structurally supports that DHp connector sequence (amino-acid composition and length) guides the handedness of the four-helix bundle [7] , [18] , [19] . The CA domains (residues 297–451) presented the characteristic α/β sandwich fold of the GHKL superfamily ( Fig. 2a ) as previously showed by NMR structure of EnvZ [20] . The DHp and CA domains were connected by a short, unstructured linker with seven residues (residues 291–296). Table 1 Diffraction data and refinement statistics for EnvZ chim . 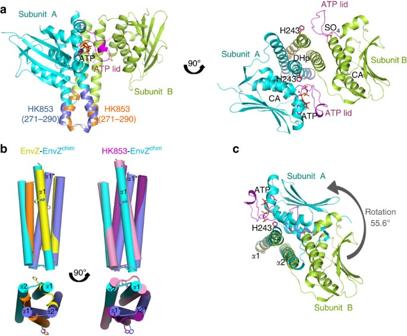Figure 2: EnvZchimstructure. (a) Overall structure of EnvZchim. Cartoon representation of the homodimeric EnvZchimstructure (subunit A in cyan and subunit B in green) in two orthogonal views. The DHp region interchanged is highlighted in blue for subunit A and in orange for subunit B. ATP lid is coloured in magenta and the AMPPNP, sulphate (SO4) and the phosphorylatable H243 are drawn as sticks. (b) Comparison of EnvZchimDHp with EnvZ and HK853. A cartoon representation, in cylindrical helices, for the DHp superimposition of homodimeric EnvZchim(one subunit in cyan and the other in blue) with EnvZ (3ZRW; one subunit in yellow and the other in orange) and HK853 (2C2A; one subunit in pink and the other in purple). In the homodimers, α-helices are labelled and phosphorylatable His are shown as sticks. Two orthogonal views, lateral and from the apex, are displayed. (c) EnvZchimstructure shows asymmetry. Superposition of DHp from subunit A (cyan) and B (green) illustrates the asymmetry due to a rotational movement of CA in relation to DHp (55.6° calculated by Dyndom). Full size table Figure 2: EnvZ chim structure. ( a ) Overall structure of EnvZ chim . Cartoon representation of the homodimeric EnvZ chim structure (subunit A in cyan and subunit B in green) in two orthogonal views. The DHp region interchanged is highlighted in blue for subunit A and in orange for subunit B. ATP lid is coloured in magenta and the AMPPNP, sulphate (SO 4 ) and the phosphorylatable H243 are drawn as sticks. ( b ) Comparison of EnvZ chim DHp with EnvZ and HK853. A cartoon representation, in cylindrical helices, for the DHp superimposition of homodimeric EnvZ chim (one subunit in cyan and the other in blue) with EnvZ (3ZRW; one subunit in yellow and the other in orange) and HK853 (2C2A; one subunit in pink and the other in purple). In the homodimers, α-helices are labelled and phosphorylatable His are shown as sticks. Two orthogonal views, lateral and from the apex, are displayed. ( c ) EnvZ chim structure shows asymmetry. Superposition of DHp from subunit A (cyan) and B (green) illustrates the asymmetry due to a rotational movement of CA in relation to DHp (55.6° calculated by Dyndom). Full size image The dimer is asymmetric, as the relative DHp-CA disposition in each subunit (named A and B) differs ( Fig. 2a,c ); however, the overall structure of the individual DHp and CA domains between A and B subunits was virtually identical except for local differences. The DHp domains in subunit A and B superimposed with an r.m.s.d. as low as 1 Å (residues 226–290), with differences localized in the N-terminal part of the α1 helix, which minimized at the level of the conserved α1 proline (Pro248). The CA domains in subunit A and B were almost indistinguishable (r.m.s.d. of 0.73 Å for the superimposition of residues 291–386 and 405–440), except for quite a different conformation of ATP lid (residues 387–404), which was probably due to a different occupancy of the ATP-binding sites. The active site of subunit A was occupied by an AMPPNP molecule ( Fig. 3a ), while subunit B contained only a sulphate ion ( Fig. 3b ), thus confirming the nucleotide conformational dependence of this region. Indeed, it is unusual to observe ATP lid in the absence of ligands, but the presence of a sulphate ion seemed to stabilize this element by interacting with the Gly401 and Thr402 ATP lid residues ( Fig. 3b ). Despite the similarity of the individual domains in both subunits, the relative disposition of their domains, and their interdomain interactions, differed considerably as a result of the CA domains’ rearrangements ( Fig. 2a,c ; Supplementary Table 1 ). In subunit B, the CA domain came close to DHp α2 helix with an orientation relative to the DHp domain more similar to that observed in other structures of HKs (HK853, PDB:3DGE; DesK, PDB:3GIE; KinB, PDB:3D36) ( Supplementary Fig. 2a ). Unlike subunit B, the CA domain from subunit A approached the α1 helix of the same subunit with an orientation that was consistent with the transfer of ATP γ-phosphate to phosphoacceptor His243 ( Figs 2a,c and 3a ), a similar disposition has been observed in the VicK subunit A (PDB:4I5S) ( Supplementary Fig. 2b ). In this conformation, the ATP molecule and the phosphorylatable His belonged to the same subunit, which structurally advanced a cis -autophosphorylation for EnvZ chim despite the trans directionality observed for EnvZ [14] , [16] . 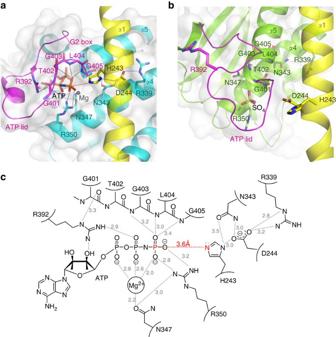Figure 3: Catalytic centre in the EnvZchimstructure. (a) Catalytic centre in subunit A. A close view in the cartoon representation showing the ATP analogue AMPPNP, phosphorylatable H243 and other relevant residues (D244, R339, N343, N347, R350, R392, G401, T402, G403, L404 and G405) as sticks. Dashed lines represent the interactions between residues and AMPPNP. ATP lid and G2 box are coloured in magenta, DHp α1 helix in yellow and CA in cyan (α4 and α5 are labelled). CA is also represented as a white semitransparent surface. (b) Catalytic centre in subunit B. A close view in the cartoon representation showing sulphate ion (SO4). Relevant residues and structural elements are shown as in (a) but the CA is in green. (c) Schematic representation of the catalytic centre in subunit A. Distances between relevant residues and the AMPPNP are indicated and drawn as dashed lines. Figure 3: Catalytic centre in the EnvZ chim structure. ( a ) Catalytic centre in subunit A. A close view in the cartoon representation showing the ATP analogue AMPPNP, phosphorylatable H243 and other relevant residues (D244, R339, N343, N347, R350, R392, G401, T402, G403, L404 and G405) as sticks. Dashed lines represent the interactions between residues and AMPPNP. ATP lid and G2 box are coloured in magenta, DHp α1 helix in yellow and CA in cyan (α4 and α5 are labelled). CA is also represented as a white semitransparent surface. ( b ) Catalytic centre in subunit B. A close view in the cartoon representation showing sulphate ion (SO 4 ). Relevant residues and structural elements are shown as in ( a ) but the CA is in green. ( c ) Schematic representation of the catalytic centre in subunit A. Distances between relevant residues and the AMPPNP are indicated and drawn as dashed lines. Full size image Catalytic centre for autophosphorylation The CA-DHp relative disposition in the subunit A showed that the AMPPNP γ-phosphate-leaving group and the His243 εN-accepting atom were at the correct distance (γP–εN 3.6 Å) and were well aligned (N AMPPNP –P–N His angle of 165°) for the catalytic reaction ( Fig. 3a,c ). Both domains contributed to form the autophosphorylation active site, but the participation of the CA domain was predominant, as it provided all the nucleotide-interacting residues, except for phosphoacceptor His243 ( Fig. 3c ). However, the DHp domain seems to play a key role since it provided Asp244, whose carboxylic side chain is bound to the δ N of His243 ( Fig. 3a,c ). This interaction allowed us to postulate that Asp244 is a general base in the reaction, as it might abstract a proton from histidine to induce its appropriate tautomeric form for the nucleophilic attack of εN to ATP γ-phosphate. This key role was supported by the conservation of an acidic amino acid at this position in the HKs ( Supplementary Fig. 3 ) and by the impaired kinase activity of the mutants at this position for several HKs [21] , [22] , [23] . At the same time, the Asp244 side chain was hydrogen bound to Asn343 and formed a salt bridge with Arg339. Triad Asn343–Asp244–Arg339 could help to achieve the correct disposition and polarization of Asp244 to act as a general base. In addition, the partially conserved Asn343 was also hydrogen bound to phosphoacceptor His ( Fig. 3a,c and Supplementary Fig. 3 ). The γ-phosphate of ATP was stabilized in the binding pocket at the correct position for the His243 nucleophilic attack, thanks to the contacts made among its three oxygens with residues from the CA domain. These contacts are with the Thr402 side chain and the backbone amide nitrogen atoms of Thr402, Gly403, Leu404 and Gly405, a helix turn that covered γ-phosphate and corresponded to the conserved HK G2 box at the beginning of helix α5 ( Fig. 3a,c and Supplementary Fig. 3 ). In subunit B, the sulphate ion, a molecule that has been reported to occupy the position of the transferred phosphoryl groups [7] , [24] , also interacted with the main chain of the first turn of helix α5 ( Fig. 3b ), thus supporting the relevance of the α5 helix dipole in γ-phosphate coordination. In addition, Arg350, placed at the end of the α4 helix, was salt bridged with γ- and β-phosphates, while Arg392 from ATP lid was salt bridged with β-phosphate ( Fig. 3a,c ). Arg350 is also hydrogen bound with Asn347 side chain, a strictly conserved asparagine in the CA domain from which the N box was named ( Fig. 3a,c and Supplementary Fig. 3 ). This Asn chelates the Mg ion required for shielding the negative charges of ATP, and it is essential for autophosphorylation [4] , [7] , [25] . Nucleotide β-phosphate also interacted with the Tyr335 side chain and the G403 main chain. Finally, α-phosphate was coordinated by the α5 helix dipole by its interaction with the backbone amide nitrogens of Leu404, Gly405 and Leu406 ( Fig. 3a ). Mutational analysis of potential catalytic residues To corroborate the autophosphorylation conformation observed in the EnvZ chim structure and to evaluate the particular contribution of each residue in the reaction, the residues involved in the interactions with phosphorylatable His and ATP γ-phosphate were individually mutated to alanine, and their catalytic activity was analysed. Furthermore, to test whether the autophosphorylation reaction was dependent of trans - or cis -directionality, we carried out this site-directed mutagenesis analysis in EnvZ and HK853. On the basis of the EnvZ chim structure, EnvZ residues Asp244, Asn343, Asn347, Arg350 and Arg392 were selected and mutated to alanine. Similarly, the structural equivalent residues in HK853, Glu261, Asn376, Asn380, Lys383 and Arg430 were mutated to alanine ( Supplementary Fig. 4 ). The autophosphorylation activity of these mutants was measured and compared with the respective wild-type forms. As an internal catalytic inactive control, the alanine mutants in the phosphoacceptor histidines of EnvZ and HK853 (His243 and His260, respectively) were evaluated. As expected, the EnvZ and HK853 His mutants showed no measurable activity, similarly to the mutants in Mg-chelating Asn (N347A in EnvZ and N380A in HK853) ( Fig. 4a ). A third mutation corresponding to the conserved acidic residue following phosphoacceptor His (Asp244 or Glu261 in EnvZ or HK853) also abolished the autophosphorylation activity in both HKs ( Fig. 4a ), which is consistent with the proposed role of the general base for this residue [3] , [13] . The mutation of the corresponding acidic residue in other HKs has a similar deleterious effect in the kinase reaction [21] , [23] . The mutation of the second residue that interacted with phosphorytable His Asn343 or Asn376 in EnvZ and HK853, respectively, also had a strong impact on both enzymes, showing residual kinase activity ( Fig. 4a ). Substituting the conserved basic residue on ATP lid (Arg392 and Arg430 for Envz and HK853) produced proteins with affected kinase activity, particularly in the case of HK853 ( Fig. 4a ). In contrast, the change in the conserved positively charged residue in the N box (Arg350 and Lys383 for EnvZ and HK853) had a modest effect, since HK853 mutant showed low kinase activity while EnvZ maintained full activity ( Fig. 4a ). 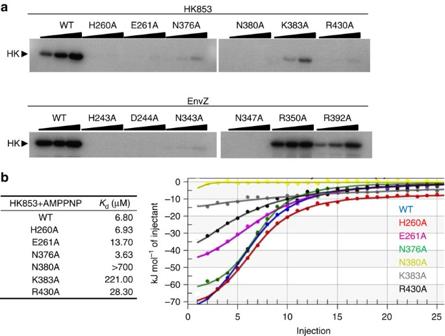Figure 4: Analysis of residues involved in the autophosphorylation catalysis. (a) Kinase assays for the wild type and mutant forms of HK853 and EnvZ. Incubation times were 2, 5 and 15 min. To facilitate the comparison, equivalent HK853 and EnvZ mutations are shown in the gels one below the other. Thus, H260A and H243A correspond to phosphorylatable His. (b) Nucleotide-biding affinity determination by ITC. The constantKd(μM) calculated for wild type and mutant forms of HK853 is shown in the table. The integrated heat responses per injection are plotted, with the solid lines representing the fit to a one-site binding model. Figure 4: Analysis of residues involved in the autophosphorylation catalysis. ( a ) Kinase assays for the wild type and mutant forms of HK853 and EnvZ. Incubation times were 2, 5 and 15 min. To facilitate the comparison, equivalent HK853 and EnvZ mutations are shown in the gels one below the other. Thus, H260A and H243A correspond to phosphorylatable His. ( b ) Nucleotide-biding affinity determination by ITC. The constant K d (μM) calculated for wild type and mutant forms of HK853 is shown in the table. The integrated heat responses per injection are plotted, with the solid lines representing the fit to a one-site binding model. Full size image With a quantitative binding assay (ITC), we tested in HK853 whether the effect produced by the mutations in the kinase reaction was purely catalytic or if it was due to a defect in the substrate binding. By using non-hydrolysable ATP analogue AMPPNP, we found that the affinity for the nucleotide ( K d =6.8 μM for the wild-type protein) was not affected by the mutations in either phosphoacceptor His ( K d =6.9 μM for the H260A mutant) or its interacting Asn376 ( K d =3.6 μM) ( Fig. 4b ). We also found that the mutation in acid residue Glu261, proposed as a general base, had a minor effect on affinity ( K d =13.7 μM) ( Fig. 4b ), which supports that both Glu261 and Asn376 residues are truly catalytic. Similarly, the mutation in ATP-lid Arg430 had only a slight effect on affinity ( K d =28.3 μM) ( Fig. 4b ). Conversely, the mutation in the conserved Asn380, which chelated Mg, abrogated the nucleotide binding entirely ( Fig. 4b ), which explained the null activity of this mutation. Substitution of Lys383 had a strong effect on nucleotide binding, which increased K d by about 40-fold (221 μM) ( Fig. 4b ). These results support an ATP-affinity role for Asn380 and Lys383, as it was previously proposed for equivalent positions in the HK PhoQ [3] . Our structural and functional results sustain a catalytic mechanism where the conserved acidic residue after phosphorylatable His acts as a general base assisted by a conserved polar residue placed in the CA domain α4 helix. Given the lower catalytic contribution observed for the positive-charged residues interacting with the nucleotide, it seems that these residues have a role in neutralizing the developed negative charge of the ADP product. Asymmetry in the autophosphorylation reaction of HK The EnvZ chim structure showed that the relative orientation of the CA domain in the ligand-bound subunit A and in the ligand-free subunit B, as compared with DHp, completely differed in each subunit, thus providing structural evidence for asymmetry in the autophosphorylation reaction ( Fig. 2a,c ). According to the Dyndom program [26] , the ligand-bound CA domain rotated 56.6° in relation to the ligand-free CA domain, inducing a closure motion of 42%, which brought the nucleotide closer to phosphoacceptor His ( Fig. 2c ). Asymmetry in the phosphorylation reaction has been biochemically demonstrated for NRII [12] and structurally predicted for DesK and VicK [9] , [11] . As we have demonstrated that EnvZ and HK853 present a similar autophosphorylation mechanism, we analysed the asymmetry of this reaction in HK853 by native electrophoresis. When HK853 was subjected to autophosphorylation in an excess of ATP (5 mM), three different species, corresponding to the un-, hemi- and bi-phosphorylated forms, were observable in native gels ( Supplementary Fig. 5 ). The time course of the reaction at 70 °C ( Thermotoga maritima optimal growing temperature) showed a fast accumulation of the hemi-phosphorylated form, which was in equilibrium with the bi-phosphorylated state when the incubation time prolonged (15–30 min). A complete HK853 bi-phosphorylation was not achieved during the time course of the reaction (90 min), but the unphosphorylated form accumulated after longer incubation times ( Supplementary Fig. 5 ). This is in close agreement with the NRII results, which showed autophosphorylation inhibition by ADP [12] . However, when ADP was removed from the media by a coupled assay with phosphoenolpyruvate and pyruvate kinase, the autophosphorylation in both subunits was complete ( Supplementary Fig. 5 ), as had been shown previously for NRII [12] . In the cell, the ATP/ADP ratio remains constant, suggesting that it is feasible that HKs always show asymmetric autophosphorylation. Therefore, the HK conformation observed in the crystal seems to represent a genuine model for autophosphorylation reaction. In addition, these results show that the asymmetry in the autophosphorylation reaction is independent of the directionality since HK853 autophosphorylates in cis [7] and NRII in trans [15] . Autophosphorylation directionality The EnvZ chim structure shows a conformation that agrees with a cis -autophosphorylation reaction, which contrasts with the trans -autophosphorylation directionality for EnvZ. To confirm that EnvZ chim cis -autophosphorylates, we analysed in vitro the reaction directionality for this chimera, as well as, the reaction directionality for HK853 chim , which was predicted to trans -autophosphorylate. HK853 and EnvZ were tested as controls. We followed the classic approach generating heterodimers formed by a short (S; cytoplasmic portion) and a long (L; cytoplasmic portion plus N-terminal tag) subunit to distinguish which subunit within the heterodimer was phosphorylated [7] , [15] . Wild type and mutants of these heterodimers were generated. The mutations impaired capacity to phosphorylate by affecting ATP binding in the long subunit (L ø ) or to be phosphorylated by eliminating phosphoacceptor His in the short subunit (S ø ) ( Fig. 5a ). The autophosphorylation of wild-type heterodimers (L/S) showed that long and short subunits were equally phosphorylated ( Fig. 5a and Supplementary Fig. 6 ); however, mutant heterodimers (L ø /S and L ø /S ø ) were differently phosphorylated in accordance with the cis or trans directionality. The mutant heterodimers of HK853 and EnvZ chim showed the same phosphorylation pattern, while HK853 chim exhibited an identical pattern to EnvZ ( Fig. 5a and Supplementary Fig. 6 ). The heterodimers HK853 and EnvZ chim carrying the mutation in the CA domain of the long subunit (L ø /S) displayed phosphorylation in the short subunit, consistently with the phosphorylation in cis, as previously demonstrated for HK853 (ref. 7 ). A double-mutant heterodimer for the CA and DHp domains in the long and short subunits (L ø /S ø ), respectively, presented no phosphorylation whatsoever, thus confirming the cis -autophosphorylation. The analogous EnvZ and HK853 chim double-mutant heterodimers (L ø /S ø ) showed phosphorylation in only the long subunit ( Fig. 5a and Supplementary Fig. 6 ), which confirmed a trans -autophosphorylation mechanism since the ATP bound in the short subunit phosphorylated the His present in the long subunit. When heterodimers EnvZ and HK853 chim presented mutations in a single subunit (L ø /S), both the long and short subunits were phosphorylated. This is explained by the spontaneous subunit exchange phenomenon that has been reported for EnvZ, which also exhibits HK853 chim [16] . As the long subunit, which was impaired to catalyse the reaction, could be phosphorylated only by the short subunit, this result also supports the trans -autophosphorylation for EnvZ and HK853 chim . Collectively, these results confirm that the EnvZ chim structure described here shows the physiological conformation of cis -autophosphorylation and that changing the connection between helices α1 and α2 in DHp is sufficient to switch the autophosphorylation directionality. 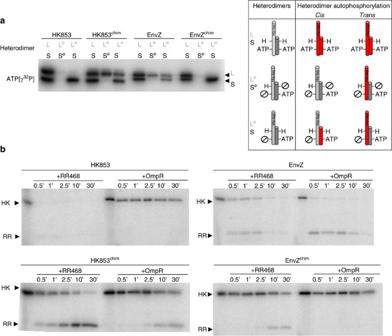Figure 5: Autophosphorylation directionality and partner recognition. (a) Autophoshorylation analysis of HK853, HK853chim, EnvZ and EnvZchimheterodimers. The heterodimers used and the possible autophosphorylation outcome are shown schematically at the right side. Heterodimers are formed by a long (L) and a short (S) form. L and S indicate the wild-type forms, Løcontains a mutation in CA (N347A for EnvZ and EnvZchim; N380A for HK853 and HK853chim) and Søcontains a mutation in phosphorylatable His (H243A in EnvZ and EnvZchim; H260A in HK853 and HK853chim). The possible phosphorylated subunits, according to acis-or atrans-directionality, are highlighted in red. In the left side is shown the electrophoretic analysis of the different heterodimers of HK853, HK853chim, EnvZ and EnvZchimby autoradiography (ATPγ32P). Autophosphorylation reaction was carried out for 10 min at 37 °C. The bands corresponding to L and S subunits are labelled. (b) Phosphotransfer capacity of HK853, HK853chim, EnvZ and EnvZchimtowards RR468 (cognate RR of HK853) and OmpR (cognate RR of EnvZ). Phosphorylated HKs were incubated with RRs for the indicated times. Bands corresponding to the HK and RR are labelled. Figure 5: Autophosphorylation directionality and partner recognition. ( a ) Autophoshorylation analysis of HK853, HK853 chim , EnvZ and EnvZ chim heterodimers. The heterodimers used and the possible autophosphorylation outcome are shown schematically at the right side. Heterodimers are formed by a long (L) and a short (S) form. L and S indicate the wild-type forms, L ø contains a mutation in CA (N347A for EnvZ and EnvZ chim ; N380A for HK853 and HK853 chim ) and S ø contains a mutation in phosphorylatable His (H243A in EnvZ and EnvZ chim ; H260A in HK853 and HK853 chim ). The possible phosphorylated subunits, according to a cis- or a trans- directionality, are highlighted in red. In the left side is shown the electrophoretic analysis of the different heterodimers of HK853, HK853 chim , EnvZ and EnvZ chim by autoradiography (ATPγ 32 P). Autophosphorylation reaction was carried out for 10 min at 37 °C. The bands corresponding to L and S subunits are labelled. ( b ) Phosphotransfer capacity of HK853, HK853 chim , EnvZ and EnvZ chim towards RR468 (cognate RR of HK853) and OmpR (cognate RR of EnvZ). Phosphorylated HKs were incubated with RRs for the indicated times. Bands corresponding to the HK and RR are labelled. Full size image Phosphotransfer specificity for chimeras The structure of the HK853–RR468 complex (PDB 3DGE) and rewiring phosphotransfer specificity experiments have shown that the DHp connector is involved in HK–RR recognition and binding ( Fig. 1b ) [7] , [27] . To assess if EnvZ chim and HK853 chim showed an altered recognition for their cognate RR (OmpR for EnvZ and RR468 for HK853) as a result of DHp connector interchange, phosphotransfer experiments were carried out ( Fig. 5b ). The results revealed that EnvZ chim lost phosphotransfer capacity to its cognate partner OmpR, but was not fully compensated by a gain of phosphotransfer to RR468. In fact, EnvZ showed a nonspecific phosphotransfer to RR468 that is dramatically reduced in EnvZ chim ( Fig. 5b ). Interestingly, HK853 chim , but not HK853, displayed a phosphotransfer to OmpR, despite long incubation times with the kinase (15 and 30 min). In parallel, HK853 chim retained the capacity to phosphotransfer to its cognate partner RR468 in a lesser extent than HK853, but it lost phosphatase activity to RR468, as observed by the accumulation of phosphorylated RR468 ( Fig. 5b ). These results confirm that the DHp area interchanged in the HKs partially overlaps with the DHp area involved in RR recognition. His/Asp phosphorylation dominates prokaryotic signalling and regulation. Stimulus sensing is initiated by autophosphorylation of HK, however, the molecular basis of this reaction is still poorly understood. Recently, the structure of VicK has shown a conformation where the CA domain approaches to the phosphoacceptor His to adopt a conformation compatible with an autophosphorylation-competent state [9] . This structure also agrees with a previous computationally derived model proposed for the autophosphorylation reaction [13] . This information has gained insights into the autophosphorylation reaction, but the absence of the nucleotide in the VicK structure has prevented a detailed analysis of the molecular basis of this reaction. The crystal structure of EnvZ chim represents the first view of the autophosphorylation reaction of a HK and has allowed us to decipher this reaction. Our structural and biochemical results have guided us to propose an autophosphorylation mechanism that is depicted in Fig. 6 . The architecture of the active centre, the geometry between the leaving and acceptor (5.3 Å and 165° from His εN to ADP O3β-phosphate) and the low positive charge stabilizing the γ-phosphate are consistent with a dissociative character for the autophosphorylation reaction [28] . In the reaction, the nucleophilic character of the phosphoacceptor His increases by the interaction with a neighboured conserved acidic residue, which is proposed to function as a base acceptor to attract the His δ N proton. The general base is assisted by a conserved polar residue placed in the CA domain α4 helix. The activated His is then polarized for in-line attack of γ-phosphate of ATP. The transfer of the phosphoryl group is facilitated and stabilized by the interaction with the Gly-rich main-chain amides of the bendable G2 box. Indeed, the introduction of rigidity into this region by mutations in the conserved Gly403 and Gly405 in EnvZ abolished kinase activity [29] . The essential Mg cation [30] plays a key role in the stabilization of the transition state, as mutations of the Mg-chelating Asn (Asn347 in EnvZ and Asn380 in HK853) entirely abolished kinase activity. Finally, the developed negative charge in the β-phosphate of the ADP product is neutralized by a conserved positive-charged residue in the ATP lid (Arg392 in EnvZ and Arg430 in HK853), as it was previously suggested for PhoQ [3] . 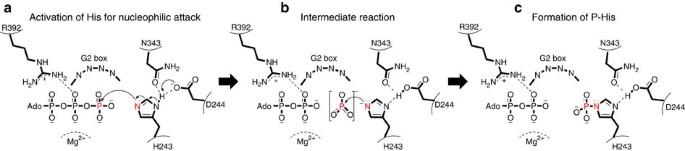Figure 6: Proposed catalytic mechanism for HK autophosphorylation. (a) Phosphoacceptor His (His243 in EnvZ) is activated for nucleophilic attack to γ-P of ATP. His nucleophilicity is enhanced by an acidic residue (D244 in EnvZ) that acts as a general base. A polar residue (N343 in EnvZ) that interacts with the general base helps to increase His nucleophilicity. γ-P of ATP is properly oriented in the binding pocket, thanks to interactions with the Gly-rich main-chain amides of the G2 box. In the intermediate reaction (b), the transfer of the phosphoryl group to the activated His is stabilized by the bendable G2 box. (c) Completion of the reaction results in the formation of P~His and the product ADP. The developed β-P negative charge in the ADP is neutralized by a positive-charged residue in the ATP lid (R392 in EnvZ) and by Mg2+cation. Figure 6: Proposed catalytic mechanism for HK autophosphorylation. ( a ) Phosphoacceptor His (His243 in EnvZ) is activated for nucleophilic attack to γ-P of ATP. His nucleophilicity is enhanced by an acidic residue (D244 in EnvZ) that acts as a general base. A polar residue (N343 in EnvZ) that interacts with the general base helps to increase His nucleophilicity. γ-P of ATP is properly oriented in the binding pocket, thanks to interactions with the Gly-rich main-chain amides of the G2 box. In the intermediate reaction ( b ), the transfer of the phosphoryl group to the activated His is stabilized by the bendable G2 box. ( c ) Completion of the reaction results in the formation of P~His and the product ADP. The developed β-P negative charge in the ADP is neutralized by a positive-charged residue in the ATP lid (R392 in EnvZ) and by Mg 2+ cation. Full size image This mechanism seems to be general for HKs, as the general base is highly conserved in HK subfamilies, HisKA (Pfam00512, 78% abundance) and HisKA_3 (Pfam07730; 12%). Indeed, the mutation of this amino acid abolishes kinase activity not only in the HKs tested herein, EnvZ and HK853, but also in several other HKs, such as CrdS, HK4262, HK1190 and NRII [21] , [23] . However, a small subset of HK subfamilies, His_kinase (Pfam06580; 7%), HisKA_2 (Pfam07568; 2%) and HWE_HK (Pfam07536; 1%), shows an invariant aromatic (His_kinase) or Arg (HisKA_2 and HWE_HK) residue at this position. Thus, an acidic residue from an alternative position should play the role of a general base in these HK subtypes. Since a polar residue in α4 interacts with the His, this position is a strong candidate to hold the alternative acidic residue. This notion is supported by the presence of an invariant Glu at this position in the HWE_HK subfamily [31] . Furthermore, members of the GHL ATPase family that share a common ATP-binding domain with HKs [5] present a conserved Glu residue at this position, which acts as a general base in the catalytic reaction [32] . The HKs’ mechanistic similarities with GHL ATPase extend to the presence of the flexible and conserved G-rich loop that stabilizes the transition state by the interaction with the main-chain amide atoms [32] , [33] . Mutations in this loop severely compromise the HK or GHL ATPase activities [29] , [34] , which supports a similar catalytic mechanism in the GHKL superfamily. The mechanism of autophosphorylation is independent of the cis - or trans -directionality since the catalytic centre in HK853 ( cis- HK) and EnvZ ( trans -HK) seems identical in accordance with our functional and structural data; thus, cis- and trans -directionality depend on the connection handedness between the DHp α1 and α2 helices. Recent in vitro observations with EnvZ and PhoR HKs also support this conclusion [19] . This connection is highly variable in sequence (both amino-acid composition and length) among HKs, therefore, the differences in the DHp connector can dictate the arrangement between the helices. The EnvZ chim structure confirms this notion since the substitution of the connector sequence of EnvZ for the corresponding portion of HK853 induces the same DHp connector handedness as HK853. But why do HKs show different connection handedness? The fact that the region interchanged in this work is involved in RR recognition, as structural (HK853–RR468 complex) [4] and functional (EnvZ rewiring) [21] data support, implies that it might be related with partner recognition specificity. Our phosphotransfer analysis of the EnvZ chim and HK853 chim showed completely altered partner selectivity, which confirms the implication of this region in RR specificity. Recent studies have demonstrated that after gene duplication the accumulation of mutations in specificity-determining residues, which encompass the DHp connector, is the major selective force in the evolution of two-component signalling pathways [35] . Therefore, it is tempting to speculate that the adaptive mutations in the sequence of this area, forced by the prevention of crosstalk between pathways after gene duplication, generate sequence combinations whose physicochemical features favour the different connection handedness to establish cis- or trans- directionality. In this way, a unique autophosphorylation mechanism imposed by a highly conserved machinery, the ATP-binding domain and phosphoacceptor His, is coupled to a variable DHp connector, which allows the flexibility required by the presence of tens to hundreds of different two-component systems in a single organism. EnvZ chim structure shows that autophosphorylation is carried out in an asymmetric way where one of the subunits is phosphorylated, while the second one is in a kinase-unproductive conformation. This asymmetry for the catalytic machinery of the HKs has been structurally confirmed by other HK structures such as DesK, VicK and YF1 (refs 8 , 9 , 11 ), where the relative disposition of DHp and CA domains is different in each subunit ( Supplementary Fig. 7 ). However, a symmetric disposition for this catalytic portion has been observed in other HKs such as HK853, ThkA, KinB or DesK [6] , [7] , [8] , [10] , [11] , [36] ( Supplementary Fig. 7 ), supporting the proposed structural plasticity of the HK catalytic machinery [11] . As in the present case, structural asymmetry in HKs has been associated with the autophosphorylation reaction [9] , [11] , whereas in all structures of HK–RR complexes the HK component is symmetric, and therefore, symmetric conformations of HKs maybe related with either phosphotransfer or phosphatase reaction [7] , [8] , [10] . In this way, the current structural knowledge is compatible with a mechanism in which the catalytic machinery of HK switches in a signal-dependent manner between an asymmetric kinase and a symmetric phosphotransfer/phosphatase-competent conformation [11] . Interestingly, the structural analysis of the sensor domains of different HKs suggests that the extracellular domains are asymmetric in the phosphatase-competent state of the HK and symmetric in the kinase-competent state [37] , [38] . Perhaps, symmetric extracellular arrangement triggers an asymmetric cytoplasmic disposition and the asymmetric extracellular arrangement triggers the symmetric intracellular disposition. Transmembrane helices or the HAMP or PAS domains that connect the extracellular sensor and intracellular catalytic modules could act as conformational switches. This notion is supported by the recently reported VicK and YF1 structures that show a dimeric HK with a symmetric arrangement of the HAMP- and PAS-regulatory domains, whereas the DHp and, specially, the CA catalytic domains are asymmetrically positioned [8] , [9] . However, it has been proposed that the specific mechanism of activation of the phosphatase reaction may differ from protein to protein, as suggested by enzymological studies with NRII, which would support that the phosphatase activity of this protein would proceed in an asymmetric conformation [39] . Cloning and mutagenesis HK853 (residues 232–489) was cloned into pET24b, as described before [6] , and into pLIC-SGC1 using ligase-independent cloning (LIC) [40] to obtain His-tag HK853. EnvZ (residues 224–450) was cloned into pET21d by the In-Fusion HD cloning technology (Clontech) and into pNIC28-Bsa4 by LIC to obtain His-tag EnvZ. EnvZ chim and HK853 chim were produced from the parental EnvZ and HK853 vectors by the In-Fusion HD cloning technology (Clontech). Site-directed mutagenesis in HK853, EnvZ, EnvZ chim and HK853 chim was performed by the Quickchange method (Stratagene). RR468 and OmpR-REC (receiver domain of OmpR; residues 1–122) containing the His tag were cloned into pNIC28-Bsa4 and pLIC_SGC1 (ref. 40 ), respectively, by LIC. The primers used for cloning and mutagenesis are presented in Supplementary Table 2 . Protein expression and purification Proteins were expressed in the BL21-codonplus(DE3)-RIL strain using 1 mM isopropylthiogalactoside at 37 °C for 3 h. EnvZ and HK853 wild type, mutants and chimeras were purified in batch by affinity chromatography using Ni 2+ magnetic beads (Sigma) following the indications of the supplier. The heterodimers were obtained by the coexpression of a protein with and without His tag and purified by affinity chromatography in a 5-ml HisTrap FF column (GE Healthcare) equilibrated with buffer A (50 mM Tris, pH 8.0 and 500 mM NaCl, pH 8.0) and eluted in a 20-column volume gradient from 0 to 30% of buffer B (buffer A plus 500 mM imidazole). The RRs OmpR-REC and RR468, containing His tag, were purified by affinity chromatography using 1-ml Histrap columns and a subsequent gel filtration in a Superdex 75 16/60 column (GE Healthcare). EnvZ chim -SeMet was obtained by in vivo labelling [41] . EnvZ chim was purified by affinity chromatography in a 5-ml HisTrap FF column equilibrated with buffer A, washed with 7.5% of buffer B and eluted with 40% of buffer B. The His tag was removed by tobacco etch virus protease digestion and the cleaved protein was purified by affinity chromatography in a HisTrap column followed by gel filtration chromatography in a Superdex 200 16/60 column. Crystallization, data collection and model building Crystals of EnvZ chim were obtained by vapour diffusion mixing 0.8 μl of protein mixture (10 mg ml −1 EnvZ chim , 4 mM AMPPNP and 4 mM MgCl 2 ) and 0.8 μl of reservoir solution (2% PEG1000, 2–6% PEG4000, 1–1.7 M (NH 4 ) 2 SO 4 , 0.1 M Hepes pH 7, 5 and 20–40 mM sodium acetate). Crystals were cryoprotected in mother liquor with increased concentrations of polyethylene glycols (PEGs) (4%, PEG1000 and 12%, PEG4000), 22% sucrose and decreased (NH 4 ) 2 SO 4 (0.85 M) concentration. Diffraction data were collected for the native crystals at Diamond Light Source I24 (Oxfordshire, UK) at 3.0 Å and for the derivative crystal containing SeMet at European Synchrotron Facility ID29 (Grenoble, France) at 3.8 Å. Data reduction of the diffraction data was performed using XDS [42] , Pointless and Scala. Phases were obtained by SIRAS using Autosol (Phenix) with the native and the SeMet-derivative data, and subsequent model building was performed with Bucanneer and Autobuild (Phenix) [43] . The final model was obtained by combining cycles of tracing (COOT) [44] and refinement (Refmac5). See Table 1 for the diffraction data statistics and the model building parameters. Pointless, Scala, Bucanneer and Refmac5 belong to CCP4 suite [45] . After refinement, the analysis of the Ramachandran plot for the EnvZ chim structure indicated that 96.8% of the residues were in favoured region, 3.24% in allowed region and 0% in disallowed region. The figures were produced using PyMOL ( http://www.pymol.org ). The movement analysis was performed with the Dyndom program [26] . Autophosphorylation assays The autophosphorylation assays were performed as previously described [46] for the indicated incubation times with minimal changes. Briefly, in general activity assays, the concentration of ATP–[γ 32 ]ATP (3000 Ci mmol −1 Perkin Elmer) was 0.1 mM–0.1 μCi μl −1 . In those assays where the catalytic mechanism was analysed (see the section ‘Mutational analysis of potential catalytic residues’), the concentration of ATP–[γ 32 ]ATP was 0.3 mM–0.1 μCi μl −1 . After reaction, samples were subjected to SDS–PAGE on 15% gel and phosphorylated proteins were visualized by phosphor imaging using a Fluoro Image Analyzer FLA-5000 (Fuji) and evaluated with the MultiGauge software (Fuji). Full gels are presented in Supplementary Fig. 8 . Phosphotransfer assays HKs were autophosphorylated with [γ 32 ]ATP at 37 °C for 10 min and phospho-HKs were loaded in a column with 0.9 ml of Sephadex G-25 fine (GE Healthcare) to remove the free ATP from the samples. Subsequently, phospho-HKs were incubated at room temperature with RR468 or OmpR-REC in equimolecular amounts for 0.5, 1, 2.5, 10 and 30 min. Phosphorylated proteins were separated, visualized and evaluated as in the previous section. Isothermal titration calorimetry The binding affinity measurements for AMPPNP and the indicated protein were taken with a Nano-ITC (TA Instruments). Experiments were carried out at 25 °C with 0.03 mM of protein in the cell and mixed with 0.7 mM nucleotide in the syringe by 30 injections of 1.5 μl each at intervals of 180 s under continuous stirring. Data integration, correction and analysis were carried out using NanoAnalyze program (TA Instruments) with a single-site binding model. Accession codes: The X-ray crystallographic coordinates reported for EnvZ chim have been deposited at the Protein Data Bank, under deposition number PDB 4KP4 . These data can be obtained free of charge via http://www.rcsb.org/pdb/home/home.do . Residues’ numbering of EnvZ chim follows the Uniprot sequence for EnvZ (P0AEJ4) and HK853 (Q9WZV7). For numbering residues of EnvZ after the HK853 insertion, we added 1,000 before the corresponding number. How to cite this article: Casino, P. et al. Visualizing autophosphorylation in histidine kinases. Nat. Commun. 5:3258 doi: 10.1038/ncomms4258 (2014).